Muscle function and hydrodynamics limit power and speed in swimming frogs Studies of the muscle force–velocity relationship and its derived n -shaped power–velocity curve offer important insights into muscular limits of performance. Given the power is maximal at 1/3 V max , geometric scaling of muscle force coupled with fluid drag force implies that this optimal muscle-shortening velocity for power cannot be maintained across the natural body-size range. Instead, muscle velocity may decrease with increasing body size, conferring a similar n -shaped power curve with body size. Here we examine swimming speed and muscle function in the aquatic frog Xenopus laevis . Swimming speed shows an n -shaped scaling relationship, peaking at 47.35 g. Further, in vitro muscle function of the ankle extensor plantaris longus also shows an optimal body mass for muscle power output (47.27 g), reflecting that of swimming speed. These findings suggest that in drag-based aquatic systems, muscle–environment interactions vary with body size, limiting both the muscle’s potential to produce power and the swimming speed. Classic studies modelling the interplay between animal speed and body size have often predicted a linear relationship between these variables [1] . Yet, the fastest animals are often neither the largest nor the smallest, but are intermediately sized, producing an n -shaped curve between speed and body mass [2] , [3] , [4] . More recent studies on terrestrial systems have suggested that this intermediate limit to sprint speed may be based on a reduced ability of limb bones and muscles to support body mass at larger sizes [5] , [6] . However, muscle power (muscle force × muscle-shortening velocity), used to propel the body forward, may also limit locomotor ability. Previous studies on terrestrial lizards have reported that muscle power may not limit sprint speed, as absolute muscle power output increases when running on greater inclines or when loaded with weights [7] , [8] , suggesting muscles are running at a submaximal power when unloaded or on level surfaces. However, the extent to which muscle power may limit speed is unclear, because we cannot easily decouple a muscle’s contribution to weight support versus propulsion. To examine muscle power limits to speed, we need to control for or remove support limitations with mass. In this regard, aquatic systems are ideal, as body mass is supported by buoyancy, removing weight support as a speed limitation. This may help determine the extent to which muscle power limits performance. The aquatic frog, Xenopus laevis , is particularly suitable for such studies, as it powers its kick almost exclusively via ankle rotation as described by Richards [9] . Thus, swimming speed is correlated to plantaris longus (PL) muscle power, which extends the ankle [10] . Similar to all muscles, this muscle is governed by two well-known properties. First, the force generated by muscle fibres depends on the instantaneous length of the sarcomeres, with maximal force occurring when the thick and thin filaments (myosin and actin) are near 100% overlap [11] . Second, the force generated by muscle fibres decreases hyperbolically as muscle-shortening velocity increases [12] . This second property can also be represented as a power–velocity curve (power=force × velocity), where power is maximal at ~1/3 of the maximum muscle-shortening velocity ( V max ), but decreases at greater and lesser velocities, producing an ‘ n -shaped’ curve. Thus, for the muscle to produce its maximal mechanical power, it must be maximally stimulated, be near 100% overlap and operate at ~1/3 V max [11] , [13] . However, below we derive a scaling model, which suggests that these criteria cannot be maintained across all body sizes, instead maximum potential muscle power may vary with body size, producing an n -shaped relationship between power and body mass (M). From our scaling model, we propose two alternative hypotheses. H 1 : muscle power limits speed. Given this limitation, we would predict an n -shaped pattern with speed and body mass for swimming frogs, similar to that reported for terrestrial animals. H 2 : factors other than muscle power limit speed. For example, if size-related bone stress is responsible for the n -shaped curve in terrestrial species, we would expect this effect to be removed for aquatic species. Thus, geometric scaling of muscle forces would predict a linear relationship between speed and body size for aquatic frogs. Here we measure the performance of swimming X. laevis , with body mass varying from 1 to 184 g and, further, we test how morphological and physiological parameters scale with body size. We show that muscle–environment interactions limit the ability of muscle to operate at 1/3 V max , predicting an ‘optimal’ body size for producing muscle power. Consequently, we show evidence for an n -shaped curve for swimming speed versus body mass. Swimming speed On the basis of our geometric scaling argument, we expected that power and, therefore, swimming speed, would follow an n -shaped trend rather than increase linearly. Supporting our hypothesis, the fastest swimming speed for X. laevis was 2.43 m s −1 observed for an intermediately sized frog of 61 g. The relationship between speed and mass was not linear, but was significantly better described by a second-order polynomial (AIC lin =−30.98, R 2 =0.46; AIC non-lin =−37.31, R 2 =0.63). This indicated an optimal mass of 47.35 g at a speed of 1.52 m s −1 ( Fig. 1b ). 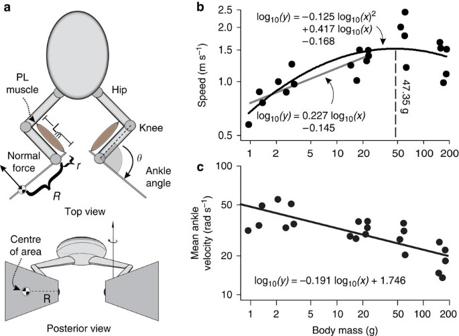Figure 1:Xenopusmodel and performance. (a) SimplifiedX. laevismodel showing the attachment of the PL muscle, the muscle in-lever (r), out-lever (R), muscle length (Lm) and ankle angle (θ). (b) Maximum swimming speed from 22 individualX. laevisversus mass showing optimum mass for speed (dashed line) from curvi-linear regression for all frogs (black line) and linear regression for small frogs (<47.35 g; grey line). (c) Mean rotational velocity of the ankle during the fastest swimming trial for each individual versus mass. Figure 1: Xenopus model and performance. ( a ) Simplified X. laevis model showing the attachment of the PL muscle, the muscle in-lever ( r ), out-lever ( R ), muscle length ( L m ) and ankle angle ( θ ). ( b ) Maximum swimming speed from 22 individual X. laevis versus mass showing optimum mass for speed (dashed line) from curvi-linear regression for all frogs (black line) and linear regression for small frogs (<47.35 g; grey line). ( c ) Mean rotational velocity of the ankle during the fastest swimming trial for each individual versus mass. Full size image Geometric scaling of morphology To further test muscle power limitations to swimming speed, we investigated the scaling of both physiological and morphological parameters. Morphological lengths of the PL muscle, tarsus and foot scaled as expected for a geometrically similar animal ( Table 1 ), supporting assumptions in the model. Similarly, consistent with previous studies [14] , in vitro muscle experiments show the scaling of , was not significantly different from M 0 ( Table 1 ). The mean for X. laevis was 6.8±0.33 L m s −1 (±s.e., n =10; Fig. 2a ). Table 1 RMA scaling exponents against mass for Xenopus laevis . 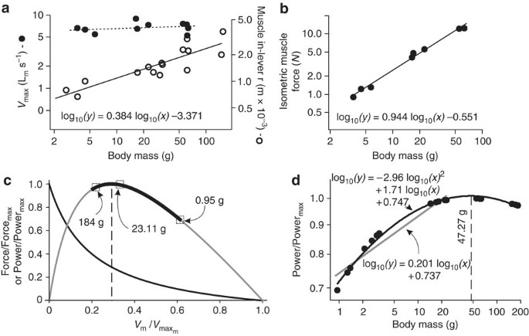Figure 2:In vitroresults forX. laevisPL muscle. (a) Maximum muscle-shortening velocity (closed circles) and in-lever (open circles) versus body mass. Dashed line indicates slope not significantly different from 0. (b) Isometric muscle force versus body mass (c) Force–velocity (thin black) and power–velocity (thin grey) curves for the PL muscle. Dashed line indicates optimal power at ~0.3Vmax. The thick black line indicates the range of maximum muscle power available for frogs based on the scaling of mean muscle velocity (Fig. 1c), arrows indicate three example body masses. (d) Maximum muscle power available from power–velocity curve (Fig. 2c) versus body mass, estimated from mean muscle velocity. Optimal mass for muscle power indicated by dashed line. Linear regression for small frogs (<47.27 g) indicated by grey line. Full size table Figure 2: In vitro results for X. laevis PL muscle. ( a ) Maximum muscle-shortening velocity (closed circles) and in-lever (open circles) versus body mass. Dashed line indicates slope not significantly different from 0. ( b ) Isometric muscle force versus body mass ( c ) Force–velocity (thin black) and power–velocity (thin grey) curves for the PL muscle. Dashed line indicates optimal power at ~0.3 V max . The thick black line indicates the range of maximum muscle power available for frogs based on the scaling of mean muscle velocity ( Fig. 1c ), arrows indicate three example body masses. ( d ) Maximum muscle power available from power–velocity curve ( Fig. 2c ) versus body mass, estimated from mean muscle velocity. Optimal mass for muscle power indicated by dashed line. Linear regression for small frogs (<47.27 g) indicated by grey line. Full size image Counter to expectations, muscle force was ∝ M 0.944 ( Fig. 2b ), significantly higher than M 0.666 predicted for a geometrically similar animal ( Table 1 ). Previously, the cross-sectional area of the PL has been shown to scale higher than expected (~M 0.9 ) due to a relatively low scaling exponent of muscle fibre length [15] . Given the positive allometry of muscle force, we modified our scaling argument to determine how muscle-shortening velocity (therefore power) must scale with mass. To balance the forces on the foot, drag force must also scale more steeply than predicted ( ∝ M 0.944 ) to balance muscle force. Substituting F drag ∝ M 0.944 in equation (4) and using geometric scaling of out-lever (R) and foot area ( A foot ) yields a predicted scaling of ankle rotational velocity ( d θ/ dt ) ∝ M −0.194 . This agrees closely with the scaling of empirical data for mean ankle rotational velocity (M −0.191 ) and maximal ankle rotational velocity (M −0.205 ) recorded in freely swimming frogs ( Table 1 and Fig. 1c ). Thus, both freely swimming frogs and in vivo data support our prediction that larger frogs rotate their ankles more slowly due to the scaling of fluid drag. Using scaling data for ankle rotational velocity, we determined the scaling of muscle-shortening velocity via measurements of in-lever and out-lever. Tendon travel experiments confirm that similar to muscle length and muscle out-lever, the scaling of the PL muscle in-lever was not significantly different from the predictions for a geometrically similar animal ( Table 1 and Fig. 2a ). Substituting ankle rotational velocity ∝ M −0.191 and r ∝ M 0.333 into equation (3), V abs should scale as M 0.142 , which is less steep than originally predicted ( ∝ M 0.33 ). As was found to be independent of body size, and muscle length scaled geometrically, should scale as M 0.333 (equation (2)). Consequently, V / V max is expected to scale as M 0.142 /M 0.333 ∝ M −0.191 , meaning that as frogs grow larger, muscles shift leftward on their power–velocity curve. Scaling of muscle power As a consequence of decreasing V / V max with body size, muscle power should trace the predicted n -shaped power curve [13] . Figure 2c shows the proportion of maximum power available to a muscle over the range of muscle-shortening velocities we have observed for frogs of different body masses (see ‘ In vivo muscle-shortening velocities’ below). When these power values for frogs are compared with body mass ( Fig. 2d ), the curve of power versus mass corresponds well to the curve for swimming speed, predicting an optimum mass with respect to power of 47.27 g, almost identical to the optimal mass predicted from swimming speeds (47.35 g; Fig. 1b ). To further compare the power–mass and speed–mass curves, we used the optimum value to separate small and large frogs. From this size-separated data, linear regression predicted a positive relationship for the speed of small frogs ( R 2 =0.72, P <0.001; analysis of variance), increasing as M 0.227 ( Fig. 1b ). The regression describing larger frogs was not significant ( R 2 =0.35, P =0.095; analysis of variance).The scaling of power with mass for small frogs was M 0.201 ( Fig. 2d ), not significantly different to that of swimming speed with mass (F 2,26 =0.490, P =0.474; Log-likelihood). Thus, the change in swimming speed with mass can be completely explained by the variation in muscle power with size. We have shown that the scaling of muscle-shortening velocity differentially limits the capacity for producing power in vitro . As muscle power is maximal at ~1/3 V max , the scaling of muscle force coupled with fluid drag force implies that this optimal shortening velocity for power cannot be reached for all body sizes, but instead follows an ‘ n -shaped’ pattern. This pattern is shown not only in our in vitro muscle results, but is mirrored in whole animal swimming speed, specifically the rate of increase of swimming speed with mass, the mass at peak swimming speed and also the subsequent decline of swimming speed with further mass increases. The correspondence between our predicted scaling for muscle power and our observed scaling for swimming speed suggests that the n -shaped power–velocity curve limits swimming speed. The n -shaped speed–mass curve predicted by our current model is in contrast to previous predictions of locomotor speed versus body size. Earlier studies suggested that as muscle force scales with cross-sectional area of the muscle, and stride frequency scales with the inverse of such, maximum speed was thought to be independent of body mass [16] . Since then, several other variations of this scaling model have predicted a positive linear relationship between speed and size [1] . In contrast with prior predictions, we have shown that at least for speed in aquatic systems, it is the interaction between a muscles power–velocity curve with stride frequency, which may ultimately limit speed and result in the observed n -shaped pattern. This muscle power limitation to swimming speed has important implications for the evolution of speed in aquatic systems. As swimming speed is often considered an ecologically relevant task for catching prey and avoiding predators, then larger body sizes may be selected against in these systems. If this scaling relationship is ecologically relevant, we may then expect to see the size distribution in natural populations centred on the optimal size for speed. Studies in wild population of Xenopus seem to support this hypothesis. Mean body size for three different reference sites in South Africa was 39 g for female frogs [17] , close to the predicted mass of 42 g, and certainly less than the maximum body size possible. The simplicity of this model suggests that these principles may be applicable to a range of animals. Most specifically, this model may be relevant for swimmers, where propulsion is ‘rowing-like’ by simple drag-based rotation, for example, in turtles [18] , aquatic insects [19] and rowing fish [20] . The model may also be extended to other species of swimming frogs [21] , although some caution should be used in that the current model only considers rotational drag. Although this is appropriate for X. laevis for which nearly 100% of the thrust is derived from rotational foot motion, in other frog species between 15–25% of the thrust may be derived from translational foot motion, suggesting multiple muscles contribute to thrust. The outcome of variation in neuro-muscular coordination of multiple muscles is unknown but is likely to be complex. For example, if the extent to which frogs generate propulsion by foot translation versus rotation shifts over body size, the scaling of swimming speed might differ from our simple model. Such effects of the scaling of limb kinematics patterns should be investigated in future work. Of additional interest beyond swimming mechanics is the degree to which this finding can be related back to terrestrial studies, which also show the n -shaped trend between maximum speed and mass. Currently, the best explanation for this trend in terrestrial systems suggests speed may increase with body size until a certain safety factor is reached, above which speed must decrease to reduce the peak forces acting on limb bones [5] , [6] , [22] . However, with increasing body size, limb beat frequency has been shown to decrease for both mammals [23] and lizards [24] , reflecting the changes in ankle rotation seen in the current study. Assuming that limb kinematics, posture and motor coordination patterns do not change dramatically over size, we would expect muscle power to similarly rise and fall as the operating point on the power–velocity curve shifts. This change in muscle power over size may then contribute to the rise and fall of speed with size in these terrestrial animals. Thus, we propose that future studies may apply our model more broadly to investigate the muscular limits of running speed. In contrast with our scaling regime, several studies on terrestrial lizards reported that power did not appear to limit speed. Power output was shown to increase as lizards ran up steeper inclines, and for animals loaded with weights [6] , [25] ; therefore, it was suggested that lizards running on level surfaces were doing so at submaximal power [7] , [8] . However, within these trials, stride frequency also varied significantly with the loading regime [7] . Along with changes in external loading, the change in stride frequency seen within these studies may have shifted the muscle along its power–velocity curve to a shortening velocity more favourable for power production, explaining changes in power output. As the current study has illustrated, performance may not be limited by maximum power output possible per se , but rather the maximum power output obtainable at a given stride frequency [26] . We have proposed a novel scaling principle predicting that relative muscle-shortening velocity ( V / V max ) decreases with body mass. For frogs, the implications of such scaling are dramatic; the negative scaling of V / V max limits power, and therefore the swimming speed. The simplicity of our model suggests that geometrically scaled drag-based swimmers, in general, are also subject to such scaling principles. For future studies, we propose that our scaling principle may more broadly apply to running animals, despite mechanical differences between land and water. Regardless of locomotor mode, muscle power may still impose a limit to speed in each case, although the constraint does not lie in the maximal ability of the muscle to produce power, but rather the ability of the muscle to produce power as the muscular–skeletal system interacts with the external environment. Scaling model Using geometric scaling principles, we show why muscles cannot produce maximum power at all body sizes. For our model, we use scaling in proportion to body mass as ∝ M b where b is the slope on a log–log plot. On the basis of geometry, we apply three scaling rules: mass (for example, muscle mass) αM 1 , length (for example, limb length) αM 1/3 and area (for example, webbed foot area) αM 2/3 . Simple models have often served to reveal general principals in complex systems [27] , [28] , [29] . We follow these examples and have modelled the movement of X. laevis as a simple muscle lever system, powered by the plantaris muscle, with a rigid flat fin rotating around about the ankle joint ( Fig. 1a ). To determine the consequences of geometric scaling on muscle function, we express ankle rotational velocity in terms of muscle-shortening velocity. Next, we determine how ankle velocity (and therefore muscle velocity) relates to propulsive drag force by rotating the feet. Our scaling argument is as follows. First, we assume that swimming animals of all sizes maximize power by maintaining V / V max =0.3. Second, we describe the scaling of foot kinematics required to satisfy the above assumption. Third, based on the scaling of fluid drag, we refute the above assumption. Fourth, we propose a more plausible scaling principle that predicts allometric scaling of V / V max , rather than geometric scaling. If muscles do produce maximum muscle power over all body sizes, we would expect all muscles to operate at a shortening velocity of 1/3 V max [13] , that is, where V rel and V abs represent the relative (muscle lengths per second, L m s −1 ) and absolute (m s −1 ) muscle-shortening velocity, respectively. For a large range of muscle types, the relative maximum shortening velocity of vertebrate muscle ( ) is nearly independent of body size [14] . If this is true for frogs, then the absolute maximum value of muscle-shortening velocity ( ) must be proportional to M 1/3 , as we can expect absolute maximum shortening velocity to be a product of relative maximum shortening velocity and muscle length, where scales as ~M 0 , whereas muscle length ( L m ) is proportional to M 1/3 for geometrically symmetrical animals [30] , leaving equation (2) αM 0 M 1/3 =M 1/3 . By substituting αM 1/3 into equation (1), we expect absolute muscle-shortening velocity ( V abs ) to also scale positively as V abs αM 1/3 to maintain V / V max αM 0 . Using this prediction for muscle-shortening velocity ( V abs ), the scaling of ankle rotational velocity is given as: where r is the muscle in-lever, θ is the ankle angle and t is time in seconds ( Fig. 1a ). As we expect muscle in-lever to scale with length as M 1/3 , we can substitute r and V abs into equation (1.3) to obtain ankle velocity αM 1/3 /M 1/3 =M 0 . Hence, to maintain V / V max =0.3 for optimal muscle power, ankle rotational velocity should be independent of body size. However, this conclusion is challenged when we consider the drag force required to move a foot through water. At high Reynolds numbers, propulsive drag ( F drag ) is proportional to the square of velocity [31] : where p is the water density, C d is the foot-drag coefficient, A foot is the foot area, R is the distance from the ankle to the fluid centre of pressure and velocity is the ankle rotational velocity. Substituting geometric scaling equations for length and area, C d αM 0 , and d θ/ dt as αM 0 predicted above, then drag force on the foot is expected to scale with positive allometry: F drag αM 0 ·M 2/3 ·(M 1/3 ·M 0 ) 2 αM 4/3 . As muscle force ( F muscle ) must resist this drag force, our assumption that all muscles operate at the peak of their power–velocity curve has created a force balance problem. Muscle force typically scales with muscle cross-sectional area [16] (αM 2/3 ), requiring that F drag also scale as M 2/3 rather than M 4/3 , to balance the forces. Therefore, R , A foot or ankle rotational velocity must scale differently to our above expectations. Given that scaling of frog hindlimbs has been shown previously [30] supporting geometric scaling for R (αM 1/3 ) and A foot (αM 2/3 ), we predict ankle rotational velocity must scale with negative allometry (that is, decrease with mass) to balance the forces. Specifically, we predict ankle rotational velocity ( d θ/ dt ) must scale as M −1/3 , enabling foot drag αM 2/3 The implication of this negative scaling of ankle rotational velocity is profound. As the body size increases, V / V max cannot be maintained at 1/3 V max where power is maximal. To summarize our scaling argument, we work backwards from equation (3). The negative allometry of ankle rotational velocity ( d θ/ dt αM −1/3 ) predicts V abs αM 0 . Consequently, αM 1/3 (equation (2)), predicting that V abs / αM −1/3 . This negative scaling of V / V max suggests that the muscles of different-sized frogs operate at different regions of their power–velocity curve, which will limit the ability of muscle to realize its maximum potential power. Consequently, we expect an n -shaped relationship between body size and maximum possible power, initially increasing until body size coincides with 1/3 V max , then decreasing as mass further increases. Animal procurement and maintenance X. laevis Daudin 1802 ( n =22, body mass range 0.95–184 g) were obtained from Xenopus Express Inc. (Plant City, FL, USA). Animals were housed in aquaria and maintained at 20–22 °C under a 12:12 h light:dark cycle, and fed twice per week. Each animal was weighed before experiments (±0.01 g) and the length of the tarsus and the foot (metatarsals+phalanges) were measured (±0.01 mm). All procedures on animals were approved by the Institutional Animal Care and Use Committee at Harvard. Swimming speed and kinematics Maximum swimming speed and kinematics for frogs<60 g were measured in a Plexiglas racetrack (15 × 180 cm) and frogs >60 g were measured in a larger tank (90 × 180 cm) at 21–22 °C. Shallow water (depth 10–12 cm) encouraged horizontal swimming. Frogs were swum down the track five to six times and filmed using a Photron Fastcam SA-3 (Photron USA Inc., CA, USA) at 250 fps. The snout tip was digitized for each trial using the MATLAB script DLTdv3 (version 3) [32] and smoothed using the spaps.m smoothing spline in MATLAB. Maximum swimming speed was calculated from the instantaneous difference between smoothed position data. Akaike’s information criterion (AIC, implemented in R (Ver 2.13.0), was used to determine whether linear or nonlinear (second-order polynomial) regressions described the relationship with speed. Measuring maximum performance across a large body size range can be difficult, as variation in body size may be correlated with variation in behavioural strategies. We therefore undertook several precautionary evaluations to ensure we were measuring maximum speeds. We have followed the advice of Losos et al . [33] who suggest that two common flaws can be seen in many published papers: data are included from individuals obviously performing submaximally and not enough trials are conducted to provide an accurate estimate of maximal capabilities. To overcome these problems, we excluded any trials where frogs failed to swim in a straight line, or hit the edges of the swim track, to remove submaximal trials. We further measured a large number of trials. We used 251 trials for 22 individual frogs (mean trials per individual=11.4), choosing the maximum speed for each individual ( Fig. 3a ). 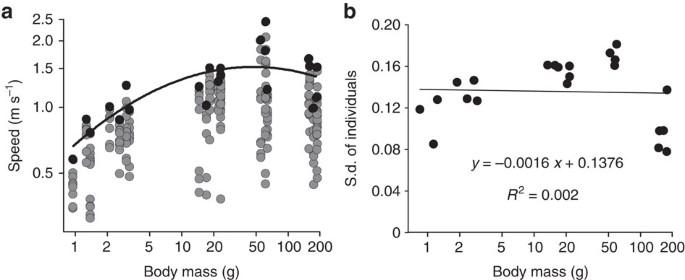Figure 3: Estimating maximum speed during swimming trials. (a) Swimming speed with mass for all trials during experimentation. Solid black circles represent maximum swim speeds for each individual, whereas grey shaded circles are submaximal swim speeds; (b) standard deviation for swimming speed with mass. Line represents the least-squares regression. Figure 3: Estimating maximum speed during swimming trials. ( a ) Swimming speed with mass for all trials during experimentation. Solid black circles represent maximum swim speeds for each individual, whereas grey shaded circles are submaximal swim speeds; ( b ) standard deviation for swimming speed with mass. Line represents the least-squares regression. Full size image We further tested the variation in submaximal trials for each body size. If swimming speed was affected by variation in behaviour, with the largest frogs showing greater variation in behaviour, we might expect that the s.d. in speeds would be highest for large frogs. This does not appear to be the case ( Fig. 3b ). The s.d. does not change consistently with body size, nor do the largest frogs show the highest variation in swim speeds, in many cases the deviation being lower than that for the smallest frogs. This suggests that large frogs are swimming close to some physical limits of their ability rather than behavioural effects. For the fastest trial for each individual, mean ankle rotational velocity (averaged over the time duration of the power stroke) was calculated from video sequences by digitizing the ankle joint, tibia and the tip of the longest toe. In vitro muscle preparation and force–velocity measurement As X. laevis swim by ankle rotation [9] , we focused on the PL muscle. We measured V max and isometric muscle force ( F o ) for a subset ( n =10) of the frogs used in the swimming trials. Frogs were double pithed with a 21-gauge syringe needle, and the PL muscle length was recorded by positioning the hip, knee, ankle and metatarsal joints at 90° and measuring the longest proportion of the muscle between the tendon and the aponeurosis. The PL was then removed, keeping the proximal attachment at the knee intact, by cutting the femur ~0.5 cm from the knee joint. Surgical suture (Vicryl 4-0, braided, Ethicon) was threaded though the femur to anchor the proximal end of the muscle. At the distal end of the PL muscle, suture was threaded through and around the PL muscle just proximal to the PL tendon. The muscle was then mounted to the ergometer, with the proximal end tied to a stiff metal pin embedded in Plexiglass, and the distal suture tied to the small hole in the lever on the servo motor (305C-LR, Aurora Scientific Inc., Aurora, ON, Canada). This setup was then bathed in oxygenated amphibian ringers solution (Carolina Biological, Burlington, NC, USA) at 22 °C. Starting tension for isotonic experimental contractions was determined experimentally using isometric twitch contractions. The passive force at which twitch muscle forces were maximal was used for starting tension. During experiments, muscle was maximally stimulated using stainless steel plate electrodes with a 150-ms pulse train at supramaximal voltage (18 V) at a spike frequency of 250 Hz based on in vivo electromyography patterns previously observed in the PL muscle of X. laevis [10] . Stimulation pulses of 1-ms width from an A/D board were amplified by an OPA549T op-amp (Texas Instruments, Dallas, TX, USA) powered by a Sorensen LS 18-5 power supply (AMETEK Programmable Power, Inc., CA, USA). The muscle was allowed to rest for 10–15 min between contractions. The isotonic force was varied in 0.1 N intervals, until the muscle was unable to move the force lever (that is, an isometric contraction), and both muscle force and muscle length were recorded with a NI-6289 data acquisition system (National Instruments, Austin, TX, USA). To calculate , the velocity of shortening ( V abs ) at each isotonic force ( F muscle ) was fitted using the equation (5), where a and b are constants specific to the muscle and F o is the maximum isometric muscle force [19] , [31] . is then calculated where the force drops to zero ( = b . F o / a ). Muscle bundle experiments To verify that our whole-muscle tissue preparations did not degrade due to the large cross-sectional area of the muscle, we performed identical experiments on muscle bundles. In the largest frogs (total body mass 105 and 168 g), we isolated muscle bundles (0.432–0.695 g in mass; ~0.1–0.2 cm 2 cross-sectional area). Under a dissecting microscope, the broad plantaris muscle was cut using a scalpel blade such that a section containing the longest fibres remained. All remaining damaged fibres were carefully removed with 2 mm spring scissors. To determine that the tissue did not degrade, we verified that the maximum tetanic isometric force remained within 10% of its initial value throughout the experiment. In addition, we verified that muscle bundles produced similar peak isometric stress (~25–30 N cm −2 ) as found in whole-muscle preparations. Finally, we compared our muscle bundle experiments to the whole-muscle results. This showed good agreement between whole-muscle experiments and muscle bundle experiments for force velocity ( Fig. 4a ) and ( Fig. 4b ). 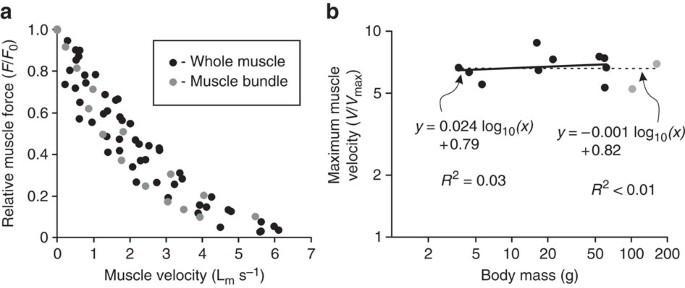Figure 4: Estimating muscle degradation with size forin vitromuscle experiments. (a) Curvi-linear relationship between relative muscle force and muscle velocity for whole-muscle preparations (solid black circles) and dissected muscle bundles (grey circles). (b) Relationship between maximum muscle velocity and mass for whole-muscle preparations (solid black circles) and dissected muscle bundles (grey circles). Solid black line is regression for whole-muscle preps, dashed line shows regression for both whole-muscle preps and muscle bundle preps combined. Results andR2shown for the solid line (left) and the dashed line (right). Figure 4: Estimating muscle degradation with size for in vitro muscle experiments. ( a ) Curvi-linear relationship between relative muscle force and muscle velocity for whole-muscle preparations (solid black circles) and dissected muscle bundles (grey circles). ( b ) Relationship between maximum muscle velocity and mass for whole-muscle preparations (solid black circles) and dissected muscle bundles (grey circles). Solid black line is regression for whole-muscle preps, dashed line shows regression for both whole-muscle preps and muscle bundle preps combined. Results and R 2 shown for the solid line (left) and the dashed line (right). Full size image Elastic energy storage To determine the extent that elastic energy storage has in this system, we re-examined data from Richards and Beiwener [10] who simultaneously measured both muscle length (using sonomicrometry crystals) and ankle angle kinematics in X. laevis . If elastic energy storage is present in the plantaris muscle, we would expect the relationship to be ‘L-shaped’, with a period showing a change in muscle length but no corresponding change in ankle angle (indicating the tendon is lengthening), and a period showing a change in ankle angle without a corresponding change in muscle length (indicating tendon recoil). This would be similar to the results shown by Astley and Roberts [34] for the vertebrate catapult in bullfrogs (see Fig. 2 in Astley and Roberts [34] ). Alternatively, if energy storage has little or no role in Xenopus swimming, we would expect a linear relationship between muscle length and ankle angle, indicating a change in muscle length corresponds directly to a change in ankle angle. 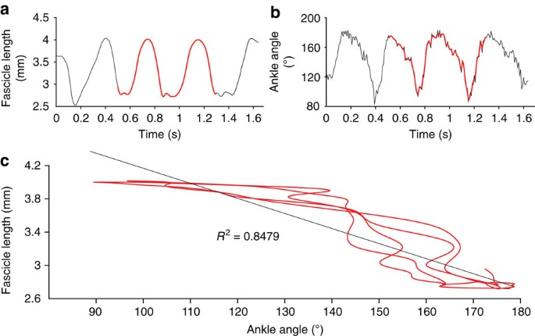Figure 5: Muscle fascicle length changes and ankle angle changes in freely swimming frogs. Data from Richard and Biewener9. (a) Time series of plantaris muscle length changes over several strokes. (b) Corresponding time series of ankle angle changes throughout the strokes. (c) Relationship between muscle length changes and ankle angle for the red highlighted sections from bothaandb. Figure 5 shows the results from the reanalysis from Richards and Beiwenier [10] , which appear to support a linear relationship between ankle angle and muscle length, suggesting little influence of elastic energy storage. Figure 5: Muscle fascicle length changes and ankle angle changes in freely swimming frogs. Data from Richard and Biewener [9] . ( a ) Time series of plantaris muscle length changes over several strokes. ( b ) Corresponding time series of ankle angle changes throughout the strokes. ( c ) Relationship between muscle length changes and ankle angle for the red highlighted sections from both a and b . Full size image In addition, evidence from mathematical modelling of a swimming limb powered by a muscle–tendon system suggests negligible effects of elastic recoil under natural conditions. Specifically, muscle–tendon simulation conditions based on X. laevis plantaris properties predict that the mechanical power contribution from the recoiling tendon does not substantially add to the power exerted by the muscle [35] . Tendon travel methods The tendon travel method was used to determine the muscle moment arm for the PL muscle. The muscle moment arm was calculated from the slope of the relationship between the length change in the PL muscle/tendon unit as the ankle joint is rotated [13] , [34] . To measure these movements, leg bones were dissected out, keeping the joint tissue at the ankle intact. The tibio-fibula was firmly attached to a surface, using suture thread, such that the flexion/extension axis was horizontal. Pins were forced into the tibio-fibula and tarsus segments to serve as markers for bone position. The proximal attachment of the PL muscle/tendon unit was severed and a long suture thread (Vicryl 4-0, braided, Ethicon) was attached to the distal end of the PL muscle. A 150-g mass was attached to the end of the suture to apply a constant load to the tendon. The foot was then flexed and extended while being filmed with a Photron fastcam (SA-3) at 250 Hz. Markers on the tarsus, tibio-fibula and the suture thread were then digitized to track displacement versus ankle angle. In vivo muscle-shortening velocities To determine the relative muscle velocity ( V rel ) for each individual, we used the mass of each individual entered into the scaling equations for mean angular velocity ( Table 1 ) and in-lever ( r ; log 10 r =0.333·log 10 mass–0.3), entered into equation (3). This was divided by muscle length as predicted from observed scaling ( Table 1 ). V / V max for each individual was then calculated by dividing through by , which was constant with mass, as 6.8 L m s −1 (see Results). Following this, muscle power for each individual could be calculated using the power–velocity curve based on Daniel [31] as shown below. Statistics All values were log 10 -transformed and scaling exponents for , F o , muscle length, in-lever, tarsus, foot length and area were determined using model II reduced major axis (RMA) regression. For each regression, the slope was tested against the expectation of isometric growth [1] . RMA slope estimates, confidence intervals and comparisons between the RMA slopes and expectations (using the likelihood ratio test) were implemented using the programme SMATR [36] . How to cite this article: Clemente, C. J. and Richards, C. Muscle function and hydrodynamics limit power and speed in swimming frogs. Nat. Commun. 4:2737 doi: 10.1038/ncomms3737 (2013).